Exploring the wavefront of hard X-ray free-electron laser radiation The high photon flux and femtosecond pulse duration of hard X-ray free-electron lasers have spurred a large variety of novel and fascinating experiments in physical, chemical and biological sciences. Many of these experiments depend fundamentally on a clean, well-defined wavefront. Here we explore the wavefront properties of hard X-ray free-electron laser radiation by means of a grating interferometer, from which we obtain shot-to-shot wavefront information with an excellent angular sensitivity on the order of ten nanoradian. The wavefront distortions introduced by optical elements are observed in-situ and under operational conditions. The source-point position and fluctuations are measured with unprecedented accuracy in longitudinal and lateral direction, both during nominal operation and as the X-ray free-electron laser is driven into saturation. The emergence of hard X-ray free-electron lasers (XFELs), such as the Linac Coherent Light Source (LCLS) [1] , [2] , has enabled many new and exciting experiments in ultrafast, high-resolution and high power-density X-ray science [3] . Among these are experiments working towards single-molecule coherent diffractive imaging [4] , [5] and time-resolved analysis of nanoscale dynamics [6] , [7] . The unique properties of XFEL radiation that enable such experiments are the pulse duration in the femtosecond range, high peak power, full lateral coherence [8] and a clean, well-defined wavefront. Hard X-ray grating interferometry, capable of recording the phase shift introduced by a sample, has found widespread application in radiography and tomography at synchrotron sources over the last decade, both in a one-dimensional [9] , [10] , [11] and, more recently, a two-dimensional implementation [12] , [13] . Recent results show that it could have a high impact in the field of biomedical imaging [14] , [15] , [16] , [17] , [18] . A grating interferometer can be used in a phase-stepping and a moiré mode, both of which are best used under different conditions. The phase-stepping mode requires the acquisition of multiple images but yields high spatial resolution and easy data processing [11] . The moiré mode, however, can provide differential wavefront information from single images, and has been shown to work for mirror metrology [19] , [20] , [21] and high-speed tomography [22] , [23] , using one-dimensional gratings, and for imaging, using two-dimensional gratings [24] . For a pulsed X-ray source like a free-electron laser (FEL), the moiré mode is preferable, and it is consequently the one we used for the measurements presented in this article. In this study, we have observed the wavefront of single shots at a hard X-ray free-electron laser. In particular, we have measured the distortions introduced by the offset mirror system, which we show to be slightly horizontally collimating and stable from shot-to-shot. Further, we have determined the shot-to-shot source-point position fluctuations in the transverse direction, as well as the source position along the beam, both during normal operation and as the FEL is driven into saturation. Grating interferometry set-up at LCLS The layout of LCLS and the grating interferometer is sketched in Fig. 1 . Electron bunches are accelerated by the linear accelerator [1] , [2] and enter the 130-m long segmented undulator, which is used to align the electrons into coherently emitting microbunches through the self-amplified spontaneous emission (SASE) process. The aligned microbunches then emit spatially coherent radiation that propagates to a pair of hard X-ray offset mirrors (HOMS) [25] . The HOMS have two important functions: they allow steering of the beam to one of the experimental stations and they effectively suppress spontaneous undulator radiation and bremsstrahlung with photon energies above 25 keV. However, they can also introduce wavefront distortions. 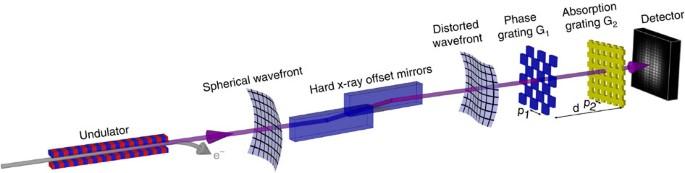Figure 1: Experimental set-up for single-shot wavefront sensing. The self-amplified spontaneous emission process in the undulator generates hard X-ray laser pulses of spherical wavefront. These pulses are filtered, steered and slightly distorted by the hard X-ray offset mirrors. The grating interferometer, located 200 m downstream of the source, consists of a checkerboard patterned silicon phase gratingG1with a period ofp1=3.991 μm and a gold absorption gratingG2with a period ofp2=2.000 μm, located at a distanced=478 mm from the phase grating. In combination, they generate a moiré pattern, from which the source location and the wavefront distortions can be extracted. Figure 1: Experimental set-up for single-shot wavefront sensing. The self-amplified spontaneous emission process in the undulator generates hard X-ray laser pulses of spherical wavefront. These pulses are filtered, steered and slightly distorted by the hard X-ray offset mirrors. The grating interferometer, located 200 m downstream of the source, consists of a checkerboard patterned silicon phase grating G 1 with a period of p 1 =3.991 μm and a gold absorption grating G 2 with a period of p 2 =2.000 μm, located at a distance d =478 mm from the phase grating. In combination, they generate a moiré pattern, from which the source location and the wavefront distortions can be extracted. Full size image About 200 m downstream of the source is the grating interferometer ( Fig. 1 ). It consists of a phase-shifting checkerboard patterned grating G 1 ( Fig. 2a ), diffracting the incident radiation and generating a mesh-shaped interference pattern downstream. The interference pattern is superimposed with a mesh-patterned absorbing analyser grating G 2 ( Fig. 2b ). The two gratings are slightly rotated with respect to each other—the superposition of interference pattern and analyser grating produces a moiré pattern ( Fig. 2c ). The analysis of such a single-shot image can deduce that the wavefront in the vertical direction is virtually distortion free, as the moiré dots follow a straight line in this direction [19] (blue line). The horizontal direction, along the HOMS reflection plane, shows some amount of wavefront distortion (red line). A distortion of one moiré fringe period corresponds to a wavefront slope error of α = p 2 /d=4 μrad, where p 2 is the analyser grating period and d the inter-grating distance. Here we observe a maximal distortion of a quarter of a fringe period, corresponding to a slope error of about 1 μrad. 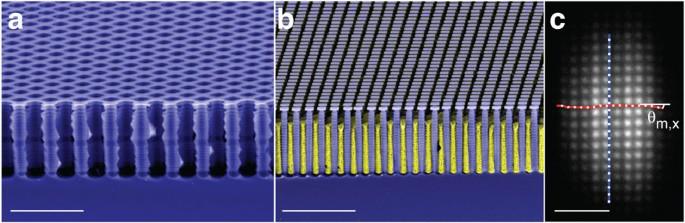Figure 2: Diffraction gratings and moiré pattern produced by their superposition. (a) Scanning electron micrograph of a cross-section through the checkerboard patterned silicon phase grating of periodp1=3.991 μm and structure heighth1=11 μm. Scale bar, 10 μm. (b) Cross-section through the mesh patterned analyser grating made of electroplated gold filled into a silicon mould. The gold structures have a period ofp2=2.000 μm and a height ofh2=7 μm. Scale bar, 10 μm. (c) Single-shot moiré pattern generated by the superposition of the interference pattern, as produced by the phase grating, with the analyser grating. From this image, one can deduce that the wavefront is distorted in horizontal direction (sketched red line) and virtually undistorted in vertical direction (sketched blue line). The average tilt of the horizontal moiré dot lines with respect to the vertical ones is due to a difference in wavefront radius of curvature. Scale bar, 250 μm. Figure 2: Diffraction gratings and moiré pattern produced by their superposition. ( a ) Scanning electron micrograph of a cross-section through the checkerboard patterned silicon phase grating of period p 1 =3.991 μm and structure height h 1 =11 μm. Scale bar, 10 μm. ( b ) Cross-section through the mesh patterned analyser grating made of electroplated gold filled into a silicon mould. The gold structures have a period of p 2 =2.000 μm and a height of h 2 =7 μm. Scale bar, 10 μm. ( c ) Single-shot moiré pattern generated by the superposition of the interference pattern, as produced by the phase grating, with the analyser grating. From this image, one can deduce that the wavefront is distorted in horizontal direction (sketched red line) and virtually undistorted in vertical direction (sketched blue line). The average tilt of the horizontal moiré dot lines with respect to the vertical ones is due to a difference in wavefront radius of curvature. Scale bar, 250 μm. Full size image Wavefront radius of curvature The wavefront radius of curvature R is related to the moiré fringe inclination angle θ m , with respect to the angle bisector between the two gratings, by where R 0 is the design radius of curvature of the interferometer (see Methods for details) and 2 β is the rotation angle between the two gratings [19] , [21] . The vertical wavefront radius of curvature is R y =190 m. This shot-to-shot wavefront measurement allows us to define the virtual longitudinal source position and its fluctuations. The observed longitudinal source position corresponds to a location about 30 m upstream of the undulator end. Because of the curvature of the HOMS, the wavefront radius of curvature in the horizontal direction is R x =362 m. The offset mirrors are slightly collimating, which could be explained by both mirrors having a radius of curvature of 800 km. This corresponds to a focal length of 275 m and a spherical mirror-profile error of 30 nm (peak to valley). The observed error is significantly larger than the spherical component of 10 nm measured ex-situ using a helium–neon laser interferometer and underlines the importance of in-situ , at-wavelength wavefront measurements. The effects of this horizontal collimation can be seen in many experiments, such as in the astigmatism observed when focussing with beryllium lenses [8] , and in the irradiance and phase profiles downstream of a simulated ideal focussing optic, as shown in the Supplementary Methods and Supplementary Figs S1, S2 and S3 . Aspheric mirror distortions To further investigate the distortions introduced by the horizontally deflecting HOMS, a grating interferometer with one-dimensional gratings and vertically oriented grating lines was installed. Although the interferometer is only sensitive along the mirror, it provides high spatial resolution, along this direction, without being limited by the moiré fringe density. The analysis of moiré patterns (see Methods ) yields the differential phase of single shots at the interferometer and, through integration, the phase profile ( Fig. 3a ) with respect to a spherical wave of radius R 0 . The largest wavefront distortions are on the order of 0.05 waves or 7 picometres, measured with a lateral resolution of 33 μm. The intensity distribution (inset, Fig. 3a ) can be extracted as well. Knowing both phase and intensity, this wavefront can be propagated to the hard X-ray offset mirror position, 43 m upstream of the interferometer. After subtraction of its spherical component, the aspherical component is projected onto the mirror to yield the aspherical component of the mirror height profile where Φ is the wavefront phase in radian, λ is the wavelength and α m =1.35 mrad is the incidence angle on the mirrors. This height profile is shown in Fig. 3b for several single shots (blue curves) and corresponds to the combined height profile of both offset mirrors. This in-situ measurement coincides nicely with the ex-situ visible light interferometer data (red curve), which had been recorded before mounting the mirrors. In addition to these higher order substrate shape errors, the X-ray grating interferometer can also observe the spherical shape error introduced by the mirror mounting, which cannot be measured using ex-situ metrology techniques. 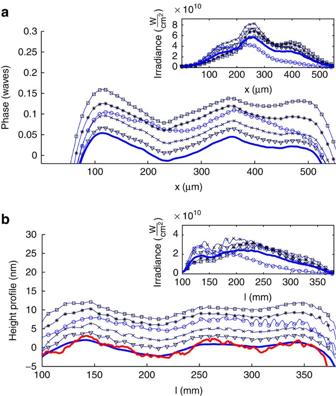Figure 3: Wavefront phase at the interferometer and height profile along both hard X-ray offset mirrors. (a) Single-shot wavefront phase at the interferometer (blue lines with markers: subsequent single shots, thick blue line: 50 shot average; the lines are plotted with 0.02 waves offset). The inset shows the corresponding irradiance profiles. (b) Combined height profile of both mirrors, aspherical component only. The single-shot wavefront information at the interferometer was propagated back to the mirror location. Projected on the mirror surface, this yields the mirror height profile. The aspherical component ofex-situvisible light interferometry measurements is plotted for comparison (red curve, seeMethodsfor details). The inset shows the corresponding irradiance profile on the mirrors. Figure 3: Wavefront phase at the interferometer and height profile along both hard X-ray offset mirrors. ( a ) Single-shot wavefront phase at the interferometer (blue lines with markers: subsequent single shots, thick blue line: 50 shot average; the lines are plotted with 0.02 waves offset). The inset shows the corresponding irradiance profiles. ( b ) Combined height profile of both mirrors, aspherical component only. The single-shot wavefront information at the interferometer was propagated back to the mirror location. Projected on the mirror surface, this yields the mirror height profile. The aspherical component of ex-situ visible light interferometry measurements is plotted for comparison (red curve, see Methods for details). The inset shows the corresponding irradiance profile on the mirrors. Full size image The irradiance profile on the mirrors varies considerably from shot-to-shot (inset, Fig. 3b ) These fluctuations are caused mainly by the pointing instability of the LCLS electron beam. For instance, the shot with blue circle markers has the same phase profile at the HOMS as all the other shots ( Fig. 3b ), but shows an exceptional irradiance profile. After propagation to the experimental station, this irradiance profile has turned into both a phase and an irradiance that differ from the other shots ( Fig. 3a ). On the order of 10% of the shots showed such an exceptional behaviour. The simulated irradiance and phase distributions downstream of an ideal, aberration-free focussing optic are shown in the Supplementary Methods and the Supplementary Figs S1–S3 , which show the same shots as Fig. 3 . Shot-to-shot source-position fluctuations To explore the shot-to-shot behaviour of the source itself in more detail, let us consider the average differential wavefront over the entire field of view of the camera. It is related to changes in lateral source position by Δ Y s = p 2 R / d ·Δ x m / p m , where Δ Y s is a change in vertical source position, Δ x m is a horizontal moiré fringe shift and p m is the fringe period. Current fringe-detection algorithms can detect shifts of 1/100th of a fringe. In combination with averaging over the entire camera image, the source-point position can be determined with an accuracy of 1–2 μm. The observed shot-to-shot fluctuation over 500 shots is 15 μm full-width at half-maximum in the vertical and 33 μm in the horizontal direction ( Fig. 4a ). It is normally distributed. The exact amount of transverse source-position fluctuation varies strongly over time, although the observed horizontal fluctuations are consistently larger than the vertical ones. The source position along the undulator, which can be observed by measuring the vertical wavefront radius of curvature R y , fluctuates by several metres ( Fig. 4b ). The longitudinal fluctuations remain stable over time. 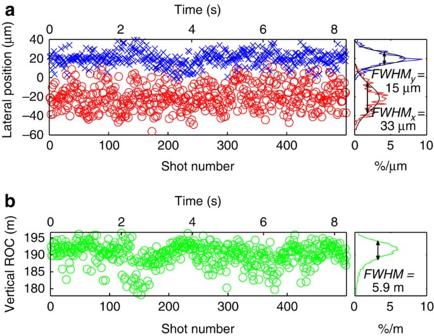Figure 4: Source-point position shot–to-shot fluctuations. (a) Vertical (blue) and horizontal (red) source-position fluctuations with their corresponding histograms. (b) Vertical wavefront radius of curvature (ROC), which is equivalent to the distance between interferometer and source point. Figure 4: Source-point position shot–to-shot fluctuations. ( a ) Vertical (blue) and horizontal (red) source-position fluctuations with their corresponding histograms. ( b ) Vertical wavefront radius of curvature (ROC), which is equivalent to the distance between interferometer and source point. Full size image Systematic source-position displacements To observe the lateral source-point position in a more systematic fashion, the electron beam along with the undulator segments was moved systematically in horizontal direction ( Fig. 5a ). Averaging 100 shots recorded at each nominal source position to reduce the influence of shot-to-shot source-point position fluctuations, the agreement between nominal and measured displacement is within 2 μm over the first four points, which confirms the expected measurement accuracy of the grating interferometer. Interestingly, one can observe not only the intentional source displacement in horizontal direction ( Fig. 5a , red curve), but also a smaller parasitic displacement of the source point in vertical direction (blue curve). 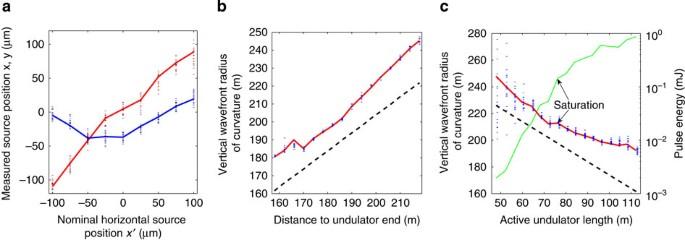Figure 5: Longitudinal and transverse source-point position. (a) Measured horizontal (red curve) and vertical (blue curve) source-point position for a nominal horizontal displacement. The solid curves show the average position of 100 shots, whereas the dashes show the position of the first 20 individual shots that were recorded at each nominal position. (b) Measured longitudinal source position. The source point was displaced in steps of 4 m by using various subsets of 13 segments out of the 28 available undulator segments (that is, segment 1 through 13, then 2 through 14, etc). Plotted is the measured wavefront radius of curvature as function of the distance between interferometer and end of the set of active undulator segments. The source point stays about two segment lengths upstream of the undulator end, which is denoted by the dashed black line. (c) Source-point position as the FEL is driven into saturation. A gain curve (green) is recorded by kicking the electron beam at different positions along the undulator. The measured radius of curvature (average shown by the red line, single shots by the blue dashes) remains about two segment lengths upstream of the kick position (black dashed line) as long as the FEL is in exponential gain regime. After the saturation point, in the linear gain regime of the FEL, the source-point distance to the end of the active undulator segments increases. Figure 5: Longitudinal and transverse source-point position. ( a ) Measured horizontal (red curve) and vertical (blue curve) source-point position for a nominal horizontal displacement. The solid curves show the average position of 100 shots, whereas the dashes show the position of the first 20 individual shots that were recorded at each nominal position. ( b ) Measured longitudinal source position. The source point was displaced in steps of 4 m by using various subsets of 13 segments out of the 28 available undulator segments (that is, segment 1 through 13, then 2 through 14, etc). Plotted is the measured wavefront radius of curvature as function of the distance between interferometer and end of the set of active undulator segments. The source point stays about two segment lengths upstream of the undulator end, which is denoted by the dashed black line. ( c ) Source-point position as the FEL is driven into saturation. A gain curve (green) is recorded by kicking the electron beam at different positions along the undulator. The measured radius of curvature (average shown by the red line, single shots by the blue dashes) remains about two segment lengths upstream of the kick position (black dashed line) as long as the FEL is in exponential gain regime. After the saturation point, in the linear gain regime of the FEL, the source-point distance to the end of the active undulator segments increases. Full size image A similar systematic experiment was performed with the longitudinal source position. Using varying subgroups of 13 subsequent undulator segments out of the total of 28 available segments, the source point was moved in well-defined steps of one undulator segment length (4 m) along the beam ( Fig. 5b ). Because of the low photon intensity produced by only 13 undulator segments, the camera integration time was increased to average over 60 shots. Despite significant photon noise, the measured wavefront radius of curvature follows the nominal displacement with an accuracy of about one undulator segment length. Throughout the experiment, the source point stays a few metres upstream of the end of the active undulator segments. The only non-smooth step in the measurement at 186 m is most likely due to a misalignment of the undulator segment that was inserted or removed at this point. Such fluctuations of the distance from the source to the undulator end reflect gain variations along the undulator. The absolute accuracy of the longitudinal source-point measurements is on the order of 4 m and the relative accuracy is 1 m. Exponential gain curve The exponential gain of a free-electron laser can be seen from the so-called gain curve ( Fig. 5c , green curve). It is obtained by kicking the electron beam from its orbit at different positions along the undulator, changing its effectively used length. LCLS has been shown to saturate after about 60 m in the hard X-ray range [1] . The grating interferometre allows us to not only measure the pulse intensity as LCLS is driven into saturation, but to simultaneously observe the source-point position along the undulator. In the exponential gain regime, before saturation, the source point follows the end of the active undulator section. From the point of saturation onwards, in the linear gain regime, the distance between measured source-point position and end of the undulator increases. In the exponential gain phase, most photons are generated on the last few metres of the undulator, because at this point the microbunching of the electrons is best. Once in saturation, the number of photons, generated per undulator segment length, remains constant—the source point is approximately at the centre between the point of saturation and the undulator end. In the low-gain region, using less than 60 m of the undulator, the radius of curvature measurements show a large spread—in this regime the single-shot measurement accuracy is limited by photon noise. For longer active undulator lengths, and especially once the FEL is saturated, the measurement quality improves considerably. We have demonstrated single-shot wavefront measurements at a hard X-ray free-electron laser. Two different types of application for this highly sensitive grating interferometry technique have been shown. We have analysed the wavefront distortions introduced by the offset mirror in-situ and under experimental conditions and we have measured the shot-to-shot fluctuations of the source-point position in the undulator, with high-resolution parallel and transverse to the direction of the undulator. This capability has been used to observe the movement in source-point position, as LCLS is driven into saturation. Grating interferometry is shown to be a valuable wavefront analysis method to understand the machine, XFEL radiation, and the performance of optical elements. Because of its moderate requirements in terms of photon flux, applications as online wavefront monitor can be envisaged using only a small, outcoupled fraction of the photon pulse without interfering with experiments taking place downstream. Grating fabrication All gratings were fabricated on silicon substrates, thinned to 30 μm thickness by deep reactive ion etching. The grating pattern was generated using an electron beam writer (Leica LION LV1) in continuous path writing mode that enables the exposure of several millimetre large gratings without introducing write-field stitching errors [26] . Because there is no easy way to record a calibration dataset, once the interferometer is installed, the accuracy of grating interferometry measurements ultimately depends on the placement accuracy of the grating structures, which is on the order of few nanometres, that is, better than 1/100th of a grating period. Grating structures fabricated for infrared coupling and filtering have been shown to have an accuracy of the average period in the sub-nanometre range [27] , [28] . Distortions introduced by the imaging system have little influence on the measurement, as it only observes moiré fringes that have large periods. The grating pattern was etched into silicon using a deep reactive ion etching process. The etch depth of the phase gratings G 1 was 11 μm, providing π phase shift at 9 keV photon energy. The absorbing analyser gratings have a gold structure height of 7 μm, absorbing more than 87% of the incident intensity. A gold layer was deposited on the trench bottom in an aluminium lift-off process analogous to the process described in ref. 29 . The trenches were subsequently filled with gold by electroplating. Experimental set-up at LCLS/XPP The experiments were performed at the X-ray pump probe (XPP) endstation of LCLS. The X-ray photon energy was set to 9 keV, corresponding to a wavelength of λ=1.4 Å, with a pulse duration of 100 fs and a pulse energy of up to 1 mJ at a repetition rate of 60 Hz. For most experiments, the beam was attenuated by an order of magnitude using silicon attenuators. The gratings were mounted in air on the LCLS/XPP sample goniometre. The inter-grating distance was set to d =478 mm corresponding to the n =33rd Talbot order of the checkerboard and line-phase gratings G 1 . They were fabricated with a period of p 1 =3.991 μm and produce an interference pattern of 2.000 μm period, when working with an R 0 =211 m distant spherical photon source. The mesh and line analyser gratings G 2 have a period of p 2 =2.000 μm. The analyser gratings were mounted on a rotation stage to enable the rotational alignment of the two gratings. Moiré fringe images were recorded using a 30 μm YAG screen imaged by a lens-coupled charge-coupled device at a frame rate of 60 Hz and 1.1 μm effective pixel size. The spatial resolution of the mirror-profile measurements is limited by the s = np 2 /2=33 μm lateral shear of the interferometer [19] , which corresponds to 25 mm when projected onto the mirror surface ( Fig. 3 ). Data processing The moiré fringe images were analysed using Fourier analysis. The method, as applied to one dimensional fringes, is described in ref. 30 . Its extension to two dimensions is straightforward, the one-dimensional Fourier transform and band-pass filters are replaced by two-dimensional ones. An iterative Gerchberg-type algorithm was implemented to reduce boundary artefacts [31] . The differential phase was unwrapped using unweighted least squares, unwrapping with a congruence operation [32] . Before propagating the wavefront ( Fig. 3 ), the one-dimensional differential phase was integrated using cumulative summing. The wave field was propagated using a transfer-function approach [33] . The distance between the two HOMS is 11 m, as an approximation the wavefront was propagated to the centre between the two mirrors, before being projected onto the mirrors. The visible light interferometer profiles of the HOMS were offset longitudinally by 30 mm, before combining them into one profile corresponding to the combined effect of both mirrors. For their precise relative position and angle, being unknown otherwise, this configuration best fits the experimental data. Retrieving absolute and quantitative values of the wavefront radius of curvature, based on equation 1, requires the camera pixels to be oriented along the angle bisector of the two gratings. Any misalignment can be compensated for by adding an offset to θ m . The camera misalignment of θ m0 =3.8 mrad was determined using a grating rotation scan, as described elsewhere [21] . How to cite this article: Rutishauser, S. et al . Exploring the wavefront of hard X-ray free-electron laser radiation. Nat. Commun. 3:947 doi: 10.1038/ncomms1950 (2012).